Divergent transcriptional activities determine limb identity Limbs develop using a common genetic programme despite widely differing morphologies. This programme is modulated by limb-restricted regulators such as hindlimb (HL) transcription factors Pitx1 and Tbx4 and the forelimb (FL) Tbx5. Both Tbx factors have been implicated in limb patterning and growth, but their relative activities and underlying mechanisms remain unclear. In this paper, we show that Tbx4 and Tbx5 harbour conserved and divergent transcriptional regulatory domains that account for their roles in limb development. In particular, both factors share an activator domain and the ability to stimulate limb growth. However, we find that Tbx4 is the primary effector of HL identity for both skeletal and muscle development; this activity relies on a repressor domain that is inactivated by a human TBX4 small-patella syndrome mutation. We propose that limb identity is largely achieved by default in FL, whereas a specific repressor activity unique to Tbx4 determines HL identity. Limbs represent a typical example of serially iterated homologous structures that share a generic programme or bauplan for their patterning and growth [1] . Indeed, a conserved genetic programme that directs limb development has emerged from studies on various species and limb structures [2] . Morphological and functional differences between forelimb (FL) and hindlimb (HL) are presumably achieved through limb-specific modulation of this generic developmental programme. Early embryological experiments indicated that anterior and posterior flank mesenchymes are stably prespecified for FL and HL limb development, respectively [3] , [4] . The molecular basis for limb-specific development remained elusive until the discovery of limb-restricted transcription factors, such as Pitx1, Tbx4 and Tbx5 [5] , [6] , [7] . Pitx1 marks posterior lateral plate mesoderm with an onset soon after gastrulation during mesoderm development (e6.5–e7.0); this expression is maintained throughout HL development [5] . On the other hand, the FL-restricted Tbx5 and HL-restricted Tbx4 are expressed just before bud outgrowth and their limb-specific expression is maintained in limb mesenchyme throughout embryonic development [6] , [7] . Although initial studies of Tbx4 and Tbx5 in chick embryos suggested that these factors contribute to limb identity [8] , [9] , further investigation in mouse embryos rather supported the view that Tbx4 and Tbx5 have equivalent functions in limbs for control of early limb bud outgrowth, but not for identity [10] , [11] , [12] , [13] , [14] . Indeed, knockout of the Tbx5 gene blocked FL bud outgrowth [11] and temporal control of this inactivation showed a narrow time dependence on Tbx5 for growth [14] . A similar narrow temporal dependence on Tbx4 was found for HL bud growth [13] , although complete knockout of Tbx4 did not prevent HL bud outgrowth as dramatically as for Tbx5 in FL [10] . Ectopic gain-of-function experiments in FL have further supported the idea that both Tbx4 and Tbx5 share growth-promoting activities [12] , an activity that is conserved in a model of an ancestral Tbx4/5 gene, as found in amphioxus [15] . Oddly, these experiments suggested that mesenchyme expression of Tbx4 and Tbx5 does not contribute to cell-autonomous skeletal patterning but that these factors are critical in a non-cell-autonomous manner for muscle and tendon patterning [16] . Whereas the relative contributions of Tbx4 and Tbx5 to limb identity remain unclear, formal evidence in support of a role of Pitx1 in specification of HL identity was provided by gene deletion in mice [17] , [18] and gain-of-function experiments in chicks [19] and mice [12] , [20] . Most significantly, the Pitx1−/− HL lose HL features and develop FL-like skeletal structures [17] , [18] . In addition to this patterning activity, Pitx1 , together with the related Pitx2 , contributes to growth of HLs [21] . These activities are conserved in evolution, as evidenced by genetic studies in sticklebacks [22] , [23] , [24] . Collectively, these studies have supported the role of Pitx1 as the upstream gene in a regulatory cascade that provides identity during HL development. As the Pitx1 mouse mutant HL is deficient in Tbx4 expression, identity and growth, and given the seemingly contradictory data on the roles of Tbx4 and Tbx5 in limb development, we devised an experimental strategy to assess the properties of each of these transcription factors in HL formation using the Pitx1−/− HL model. We now provide evidence that Tbx4 and Tbx5 share both the capacity to rescue Pitx1−/− HL growth and an activator domain that correlates with this growth-promoting activity. Further, we show that only Tbx4 can rescue HL skeletal and muscle patterning, thus identifying Tbx4 as the primary effector of HL identity. This patterning activity is correlated with a transcriptional repressor domain only found in Tbx4 and that is inactivated by the human small-patella syndrome mutation TBX4Q531R . Although Pitx1 may be considered as the master regulator for specification of HL identity, this study work clearly defines Tbx4 as the downstream effector functioning on the limb generic programme to determine HL specificity. Tbx4 not Tbx5 rescues Pitx1-dependent HL morphology Because Pitx1 controls the expression of Tbx4 [17] , [19] , it has been difficult to assign their respective roles in the HL developmental programme. We used the Pitx1-deficient HL to define the growth and patterning properties of Tbx4 and Tbx5 . We first assessed the reduction of Tbx4 expression in Pitx−/− HL, at the levels of both RNA by whole-mount in situ hybridization ( Fig. 1a ) and protein by immunohistochemistry ( Fig. 1b ) and western blot ( Fig. 1c ). The data showed a reduction in Tbx4 expression of about fourfold in e11.5 HL buds. We used limb-specific Prx1-Tbx4 or Prx1-Tbx5 transgenes ( Fig. 1d,e ) to achieve expression levels that are similar to normal HL levels of Tbx4, as assessed by reverse transcriptase quantitative PCR ( Fig. 1f ). Thus, the restoration of Tbx4 expression in Pitx1−/− mutant HL provided a test of Tbx4's ability to confer HL properties in its normal developmental context. 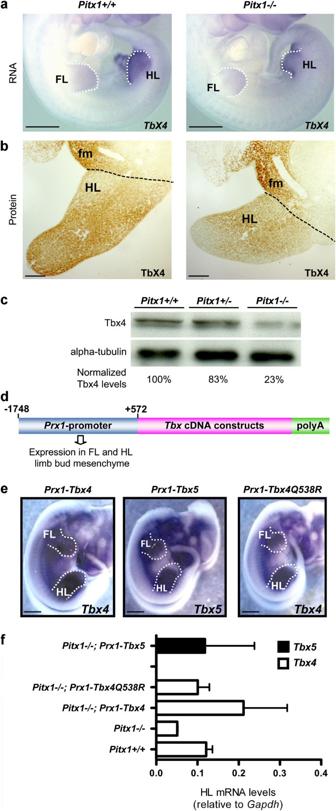Figure 1: Rescue ofTbx4expression inPitx1−/−hindlimb buds. (a)In situhybridization showingTbx4mRNA expression in wild-type (Pitx1+/+) andPitx1−/−e10.5 HL buds. Bar represents 500 μm. (b) Immunohistochemical detection of nuclear Tbx4 protein in transverse sections of e11.5 embryos of wild-type andPitx1−/−HL buds and flank mesenchyme (fm). Bar represents 100 μm. (c) Western blot analysis of Tbx4 and α-tubulin levels inPitx1+/+,Pitx1+/−andPitx1−/−e11.5 HL buds. Normalized Tbx4 levels are shown relative to α-tubulin levels (n=3). (d) Schematic representation of transgenes used in this study. Transgenic activity of thePrx1promoter was described previously37. (e) Whole-mountin situhybridization analysis of transgene expression in e11.5 embryos. Bar represents 500 μm. (f) Quantitation ofTbx4,Tbx5orTbx4Q538Rexpression levels by reverse transcriptase–quantitative PCR performed on RNA extracted from dissected e11.5 HL buds expressed relative toGapdhmRNA. Error bars indicate s.e.m. (n=3). Figure 1: Rescue of Tbx4 expression in Pitx1−/− hindlimb buds. ( a ) In situ hybridization showing Tbx4 mRNA expression in wild-type ( Pitx1+/+ ) and Pitx1−/− e10.5 HL buds. Bar represents 500 μm. ( b ) Immunohistochemical detection of nuclear Tbx4 protein in transverse sections of e11.5 embryos of wild-type and Pitx1−/− HL buds and flank mesenchyme (fm). Bar represents 100 μm. ( c ) Western blot analysis of Tbx4 and α-tubulin levels in Pitx1+/+ , Pitx1+/− and Pitx1−/− e11.5 HL buds. Normalized Tbx4 levels are shown relative to α-tubulin levels ( n =3). ( d ) Schematic representation of transgenes used in this study. Transgenic activity of the Prx1 promoter was described previously [37] . ( e ) Whole-mount in situ hybridization analysis of transgene expression in e11.5 embryos. Bar represents 500 μm. ( f ) Quantitation of Tbx4 , Tbx5 or Tbx4Q538R expression levels by reverse transcriptase–quantitative PCR performed on RNA extracted from dissected e11.5 HL buds expressed relative to Gapdh mRNA. Error bars indicate s.e.m. ( n =3). Full size image The Pitx1−/− mutant HLs lose a number of HL skeletal features, undergo HL-to-FL-like transformations, gain one FL-like feature and exhibit growth defects. We observed overall Tbx4 rescue of HL skeletal features that are dependent on Pitx1 , such as pelvic girdle and general HL morphology ( Fig. 2 , column 3 compared with 1, 2). Pitx1−/− HLs do not develop the ilium and this results in anterior displacement of the limbs: both defects were rescued by Tbx4 ( Fig. 2a–c ). Another hallmark of HLs is the rotation of limbs from a lateral to a ventromedial position: this rotation is not observed in the absence of Pitx1 and it was rescued by Tbx4 ( Fig. 2a ). Bone contacts of Pitx1−/− knee joints represent the most striking HL-to-FL-like transformation [17] , [18] . In Pitx1−/− HL, the fibula switches contacts from tibia to femur ( Fig. 2d,e , column 2) similar to the FL joint. Proper knee contacts were re-established in the Tbx4-rescued HL and the head of the fibula seemed to be 'repulsed' away from the femur ( Fig. 2d,e , column 4). At the distal joint, Tbx4 expression restored the normal angle of the calcaneus relative to footplate in Pitx1−/− HL ( Fig. 2f ). Finally, the HL programme also seems to include suppression of one FL feature, namely, the deltoid tuberosity of the humerus ( Fig. 2g , column 5), for which there is no HL counterpart. A similar tuberosity is observed on Pitx1−/− femurs ( Fig. 2g , column 2) and it was always suppressed in Tbx4-rescued HL ( Fig. 2g , column 3). Interestingly, two HL features lost in Pitx1−/− embryos, namely, the patella and small fibula/tibia width ratio, were not rescued by Tbx4 ( Fig. 2a,d ). The simplest interpretation is that these features require either Pitx1 itself or another Pitx1 target gene different from Tbx4 . In summary, Tbx4 rescued the bulk of skeletal defects associated with the Pitx1−/− loss of HL identity. 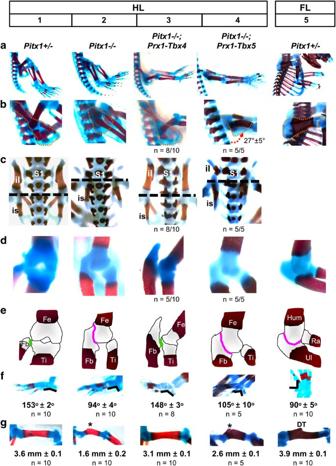Figure 2: Rescue ofPitx1−/−HL skeletal defects byTbx4but notTbx5. (a) Lateral view of e17.5 skeletal preparations (alcian blue/alizarin red staining of cartilage and bone, respectively) showing lower spine and HL ofPitx1+/−(identical toPitx1+/+),Pitx1−/−and transgene rescues. (b) Angle of pelvis (dotted outline) relative to spine. The increased angle observed inTbx5transgenics (column 4) was quantitated (± s.e.m.) in embryos showing displacement (n=5/5). FL scapula (dotted line) relative to spine angle in column 5. (c) Loss of ilium (il) inPitx1−/−(column 2) embryos and anterior HL displacement with femur head aligned (dotted line) with sacral vertebra S1 rather than S3 (column 1). Complete rescue of ilium and HL position in 8 of 10 (partial in 2)Tbx4transgenic mice (column 3), but not inTbx5transgenic mice (n=5/5). Is, ischium. (d) Limb joints for indicated limb and genotype. (e) Schematic of bone contacts, with green line between fibula (Fb)/tibia (Ti) inPitx1+/−andPitx1−/−;Prx1-Tbx4HL and magenta between ulna (Ul)/humerus (Hum) in FL or mutant fibula/femur (Fe) inPitx1−/−mutant andPitx1−/−;Prx1-Tbx5HL. Rescue of normal HL contacts in 5 of 10Tbx4transgenic skeletons examined (column 3), but not inTbx5(n=5/5). (f) Angle (black line) between calcaneus and footplate in HL or between pisiform and handplate in FL. Angle (± s.e.m.) measured for the number (n) of rescued embryos as indicated. (g) Femur length (± s.e.m.) for indicated genotypes and number (n) of embryos examined.Pitx1−/−femurs develop a tuberosity (asterisk, columns 2 and 4) that is similar to humerus deltoid tuberosity (DT, column 5). Figure 2: Rescue of Pitx1−/− HL skeletal defects by Tbx4 but not Tbx5 . ( a ) Lateral view of e17.5 skeletal preparations (alcian blue/alizarin red staining of cartilage and bone, respectively) showing lower spine and HL of Pitx1+/− (identical to Pitx1+/+ ), Pitx1−/− and transgene rescues. ( b ) Angle of pelvis (dotted outline) relative to spine. The increased angle observed in Tbx5 transgenics (column 4) was quantitated (± s.e.m.) in embryos showing displacement ( n =5/5). FL scapula (dotted line) relative to spine angle in column 5. ( c ) Loss of ilium (il) in Pitx1−/− (column 2) embryos and anterior HL displacement with femur head aligned (dotted line) with sacral vertebra S1 rather than S3 (column 1). Complete rescue of ilium and HL position in 8 of 10 (partial in 2) Tbx4 transgenic mice (column 3), but not in Tbx5 transgenic mice ( n =5/5). Is, ischium. ( d ) Limb joints for indicated limb and genotype. ( e ) Schematic of bone contacts, with green line between fibula (Fb)/tibia (Ti) in Pitx1+/− and Pitx1−/− ; Prx1-Tbx4 HL and magenta between ulna (Ul)/humerus (Hum) in FL or mutant fibula/femur (Fe) in Pitx1−/− mutant and Pitx1−/− ; Prx1-Tbx5 HL. Rescue of normal HL contacts in 5 of 10 Tbx4 transgenic skeletons examined (column 3), but not in Tbx5 ( n =5/5). ( f ) Angle (black line) between calcaneus and footplate in HL or between pisiform and handplate in FL. Angle (± s.e.m.) measured for the number ( n ) of rescued embryos as indicated. ( g ) Femur length (± s.e.m.) for indicated genotypes and number ( n ) of embryos examined. Pitx1−/− femurs develop a tuberosity (asterisk, columns 2 and 4) that is similar to humerus deltoid tuberosity (DT, column 5). Full size image In contrast, the Tbx5 transgene was unable to rescue the Pitx1−/− HL patterning defects ( Fig. 2c–g , column 4), despite being expressed at similar levels compared with the Tbx4 transgene ( Fig. 1f ). However, introduction of Tbx5 in Pitx1−/− HL produced one novel skeletal transformation that is reminiscent of an FL-specific feature: indeed, the angle of the pelvic girdle relative to spine in Tbx5 transgenics is greater (by 27°±5°) than normal, Pitx1−/− and Tbx4 -rescued pelvic girdles ( Fig. 2b , column 4 versus 1, 2, 3) reminiscent of the scapula/spine angle ( Fig. 2b , column 5). However, the ability of Tbx5 to direct the appearance of FL features in HL may be limited by the assay as it relies on expression at an ectopic site. These data unambiguously highlight the unique HL determination properties of Tbx4 and suggest limited FL determination activity for Tbx5 . Tbx4 but not Tbx5 rescues HL muscle patterning Both Pitx1 [20] and Tbx4/Tbx5 [16] have been suggested to contribute to muscle and tendon patterning. We assessed muscle patterning in e14.5 HL of Pitx1+/+ , Pitx1−/− and Tbx4 or Tbx5 expressing mutant HLs using whole-mount in situ immunohistochemistry against myosin heavy chain (MHC) ( Fig. 3a–d, g–j ), and identified individual muscles using optical projection tomography [25] , [26] images of normal limbs ( Fig. 3e,f,k,l ). A characteristic feature of HL zeugopod anterior muscles is their attachment to skeletal elements at or below the knee joint ( Fig. 3a,g ). In Pitx1−/− HL, these muscles are displaced proximally ( Fig. 3b ) such that they now reach the level of stylopod muscles ( Fig. 3b,h ). Tbx4 fully rescued the position of these muscles ( Fig. 3c,i ), but not Tbx5 ( Fig. 3d,j ). These muscles take part in control of movement by autopod skeletal elements; in HL, this control is thus independent of stylopod structures (except for the extensor digitorum longus, Fig. 3e ). This is in sharp contrast to FL, in which equivalent muscles reach from stylopod to autopod, thus providing a finer coordination of autopod movements ( Fig. 3f ). The proximal shift of these muscles observed in Pitx1−/− HL therefore represents a transformation that renders muscle patterning more similar to an FL pattern [27] ( Fig. 3f ). Ectopic expression of Pitx1 in FL [20] was shown to change the split extensor carpi radialis muscles into a single muscle similar to the HL tibialis anterior (TA, Fig. 3e,f ). In agreement with these observations, Pitx1−/− TA is split into two muscles ( Fig. 3b ) similar to FL extensor carpi radialis, and Tbx4 expression restored normal TA morphology ( Fig. 3c,i ). Another striking transformation is observed for the extensor digitorum brevis that normally links the calcaneus to phalanges within the autopod ( Fig. 3a,e ); in FL, the corresponding muscle [28] , the extensor indicus propius (EIP), reaches out of the autopod to attach to the ulna ( Fig. 3f ). Interestingly, the extensor digitorum brevis seems to be displaced proximally from the autopod to the zeugopod in Pitx1−/− HL ( Fig. 3b ) and this is rescued by Tbx4 ( Fig. 3c ). It is noteworthy that ectopic overexpression of Pitx1 in FL led to a reciprocal transformation, that is, a distal shift of the extensor indicus propius [20] . Collectively, the data support the role of Tbx4 in HL-specific patterning of both skeleton and muscles ( Table 1 ). 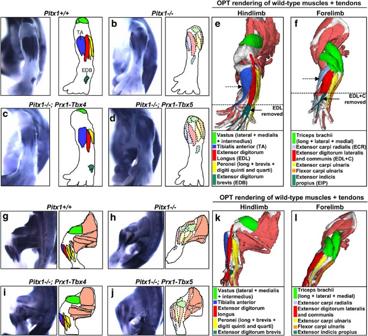Figure 3:Tbx4rescues muscle patterning ofPitx1−/−hindlimbs. Front (a–d) and lateral (g–j) views of hindlimbs from e14.5 embryos stained by whole-mount immunohistochemistry for myosin heavy chain. The lower leg (zeugopod) muscles of (a,g)Pitx1+/+, (b,h)Pitx1−/−, (c,i)Pitx1−/−;Prx1-Tbx4and (d,j)Pitx1−/−;Prx1-Tbx5HL are highlighted and colour coded in the drawings. Lighter colours inb,d,handjreflect muscle assignment by analogy in mutants with altered patterning. (e,f) Optical projection tomography (OPT) of wild-type e14.5 (e) HL and (f) FL muscles is depicted by colour-coded identification. In the lower part below the dotted line, EDL or EDL+C was removed to visualize the underlying EDB or EIP. (k,l) Lateral OPT views of HL and FL. Dotted arrows indicate TA (e) and ECR (f), whereas full arrows point to EDB (in HL,e) and EIP (in FL,f). Analogy between HL and FL muscles is based on comparative studies28,39. OPT pictures were generated using J Atlas View (http://www.nimr.mrc.ac.uk/3dlimb/)25,26. Figure 3: Tbx4 rescues muscle patterning of Pitx1−/− hindlimbs. Front ( a – d ) and lateral ( g – j ) views of hindlimbs from e14.5 embryos stained by whole-mount immunohistochemistry for myosin heavy chain. The lower leg (zeugopod) muscles of ( a , g ) Pitx1+/+ , ( b , h ) Pitx1−/− , ( c , i ) Pitx1−/− ; Prx1-Tbx4 and ( d , j ) Pitx1−/− ; Prx1-Tbx5 HL are highlighted and colour coded in the drawings. Lighter colours in b , d , h and j reflect muscle assignment by analogy in mutants with altered patterning. ( e , f ) Optical projection tomography (OPT) of wild-type e14.5 ( e ) HL and ( f ) FL muscles is depicted by colour-coded identification. In the lower part below the dotted line, EDL or EDL+C was removed to visualize the underlying EDB or EIP. ( k , l ) Lateral OPT views of HL and FL. Dotted arrows indicate TA ( e ) and ECR ( f ), whereas full arrows point to EDB (in HL, e ) and EIP (in FL, f ). Analogy between HL and FL muscles is based on comparative studies [28] , [39] . OPT pictures were generated using J Atlas View ( http://www.nimr.mrc.ac.uk/3dlimb/ ) [25] , [26] . Full size image Table 1 Summary of Pitx1−/− hindlimb (HL) defects and rescue by Tbx4 , Tbx5 and Tbx4Q538R . Full size table Growth properties shared by Tbx4 and Tbx5 The Tbx4 and Tbx5 have been implicated in the regulation of early limb bud growth and bone length [11] , [12] , [13] , [29] . We thus assessed the ability of Tbx4 and Tbx5 to restore skeletal growth defects in Pitx1−/− HL. Tbx4 rescued femur length in Pitx1-deficient HL and Tbx5 was almost as effective ( Fig. 2g , columns 3 and 4 versus 2). Interestingly, both Tbx factors rescued the left–right asymmetry in femur length [21] observed in Pitx1−/− HL ( Fig. 4a ). Another bone length defect is reflected by the HL fibula/tibia length ratio. This ratio reflects both altered growth and patterning difference at the HL compared with those at the FL stylopod/zeugopod junction. This ratio is increased in Pitx1−/− HL and becomes similar to the length ratio of FL ulna/radius ( Fig. 4b ). Tbx4 and Tbx5 transgenes decreased this ratio significantly, although less so for Tbx5 and not reaching the wild-type HL ratio ( Fig. 4b ). These data confirm the shared growth-promoting activity of Tbx4 and Tbx5, in agreement with previous gain-of-function experiments in FL buds [12] . Indeed, although Tbx4 can substitute for Tbx5 to support FL development [12] , Tbx5 is not equivalent to Tbx4 to dictate the HL programme ( Table 1 ). Collectively, these data suggest that the generic or default limb development programme depends on shared activities of Tbx4 and Tbx5 and the present data clearly defined Tbx4-dependent HL-specific skeletal patterning mechanisms. 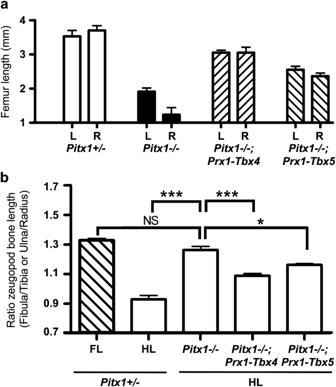Figure 4: Rescue ofPitx1−/−HL bone growth byTbx4andTbx5expression. (a) Length (± s.e.m.,n=5–10) of left (L) and right (R) femurs for skeletons of indicated genotypes. (b) Ratio of zeugopod bone lengths in limbs of indicated genotypes. ***P<0.01, *P<0.05 and NS, not significant. Error bars indicate s.e.m. (n=5–10). Figure 4: Rescue of Pitx1−/− HL bone growth by Tbx4 and Tbx5 expression. ( a ) Length (± s.e.m., n =5–10) of left (L) and right (R) femurs for skeletons of indicated genotypes. ( b ) Ratio of zeugopod bone lengths in limbs of indicated genotypes. *** P <0.01, * P <0.05 and NS, not significant. Error bars indicate s.e.m. ( n =5–10). Full size image Molecular mechanism underlying HL-specific activity of Tbx4 To investigate the molecular basis of shared and unique activities of Tbx4 and Tbx5, we assessed their transcriptional properties in cells transfected with luciferase reporters containing either monomer or dimer of T-box-binding elements (TBE). As previously reported, Tbx5 functioned as a transcriptional activator [30] , whereas Tbx4 repressed these reporters ( Fig. 5a ). Both activator and repressor activities were mapped to C-terminal domains using Gal4DBD chimeras ( Fig. 5b,d ). Deletion mapping located the Tbx5 activator domain to its distal C-terminus ( Fig. 5b , green box) in agreement with previous reports [30] . In contrast, the Tbx4 C-terminus contains a repressor domain ( Fig. 5b , magenta box in construct 6) but its deletion resulted in unmasking an activator domain that was lost on further deletion ( Fig. 5b , green box in construct 7). These data suggest that Tbx4 is unique by having a repressor domain not shared with Tbx5. It also contains an activator domain that exhibits 49% sequence conservation compared with Tbx5 ( Fig. S1a,b ). It is thus reasonable to propose that the HL-specific activities of Tbx4 may correlate with its repressor activity, whereas the growth stimulatory activities shared with Tbx5 may be ascribed to the conserved activator domain. 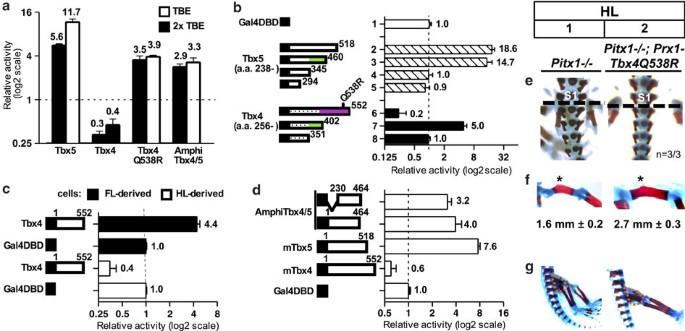Figure 5: Hindlimb-specific functions of Tbx4 correlate with repressor activity that is lost in human small-patella mutationTBX4Q531R. (a) Transcriptional activities of mouse Tbx5, Tbx4, Tbx4Q538R and amphioxus Tbx4/5 in CV-1 cells assessed with reporter containing T-box-binding regulatory element (TBE) in one or two copies (2× TBE). Error bars indicate s.e.m. (n=5) (b) Deletion analysis of Tbx4/Tbx5 C-terminal domains using Gal4DBD fusions. Deletion end points are indicated in diagrams. Green box indicates the activator domain, whereas magenta box represents the repressor domain. Error bars indicate s.e.m. (n=5). (c) Tbx4 is a transcription activator in e11.5 FL primary cells and a repressor in HL primary cells. The activity of full-length Tbx4 fused to Gal4DBD was assessed by transfection in primary cells of indicated limb buds. Data are represented as means ± s.e.m. (n=3). (d) Full-length amphioxus Tbx4/5 and its C-terminus have activator properties in CV-1 cells transfected as inbabove. Error bars indicate s.e.m. (n=3). (e–g) TheTbx4Q538Rtransgene is unable to rescue (e) ilium development and HL anterior displacement (dotted line) (f) to suppress ectopic tuberosity (asterisk) or (g) change pelvic angle, but rescues femur length (± s.e.m.,n=3). Alizarin red and alcian blue staining was carried out as shown inFigure 2. Figure 5: Hindlimb-specific functions of Tbx4 correlate with repressor activity that is lost in human small-patella mutation TBX4Q531R . ( a ) Transcriptional activities of mouse Tbx5, Tbx4, Tbx4Q538R and amphioxus Tbx4/5 in CV-1 cells assessed with reporter containing T-box-binding regulatory element (TBE) in one or two copies (2× TBE). Error bars indicate s.e.m. ( n =5) ( b ) Deletion analysis of Tbx4/Tbx5 C-terminal domains using Gal4DBD fusions. Deletion end points are indicated in diagrams. Green box indicates the activator domain, whereas magenta box represents the repressor domain. Error bars indicate s.e.m. ( n =5). ( c ) Tbx4 is a transcription activator in e11.5 FL primary cells and a repressor in HL primary cells. The activity of full-length Tbx4 fused to Gal4DBD was assessed by transfection in primary cells of indicated limb buds. Data are represented as means ± s.e.m. ( n =3). ( d ) Full-length amphioxus Tbx4/5 and its C-terminus have activator properties in CV-1 cells transfected as in b above. Error bars indicate s.e.m. ( n =3). ( e – g ) The Tbx4Q538R transgene is unable to rescue ( e ) ilium development and HL anterior displacement (dotted line) ( f ) to suppress ectopic tuberosity (asterisk) or ( g ) change pelvic angle, but rescues femur length (± s.e.m., n =3). Alizarin red and alcian blue staining was carried out as shown in Figure 2 . Full size image The Tbx4 HL patterning activity revealed in this study sharply contrasts the lack of any such activity in previous studies in which Tbx4 was overexpressed in FL [12] . A simple explanation for this discrepancy might be that the FL and HL mesenchymes have different properties in agreement with cell aggregation experiments [31] . For example, the presence of an HL-specific transcriptional co-repressor functioning with Tbx4 could fully support this model, as was documented in other systems [32] , [33] . We directly assessed the transcriptional properties of full-length Tbx4 in primary cultures derived from mouse e11.5 HL and FL buds ( Fig. 5c ). These experiments clearly showed the ability of HL-derived cells to support the repressor activity of Tbx4. In striking contrast, Tbx4 did not exhibit any repressor activity in FL-derived cells, but rather behaved as a transcriptional activator ( Fig. 5c ). These data reconcile our observations with the ectopic gain-of-function experiments performed by overexpression in FL: clearly, FL-derived mesenchyme cannot support the relevant Tbx4 HL-specifying activity. Tbx4 repressor activity correlates with HL patterning It is noteworthy that dominant human mutations of TBX4 cause small-patella syndrome, a congenital malformation affecting HLs [34] . The TBX4Q531R (mouse Tbx4Q538R ) small-patella mutation maps within the Tbx4 repressor domain ( Fig. 5b ) and we observed that this mutant protein lost repressor but retained activator functions ( Fig. 5a ). Consistent with the loss of repressor activity, Tbx4Q538R failed to rescue HL-specific features, including formation of the ilium and anterior HL displacement, knee joint and calcaneus structure ( Fig. 5e–g ), and also failed to suppress ectopic femoral tuberosity ( Fig. 5f ). In contrast, Tbx4Q538R is as efficient as Tbx4 and Tbx5 for rescue of femur length ( Figs 2g and 5f ). Finally, this mutant did not change the angle between pelvic girdle and spine and is thus devoid of this Tbx5-specific FL property ( Fig. 5g ). In summary, the Tbx4Q538R mutant is only deficient in its ability to direct HL-specific features while retaining the shared Tbx4/5 property to stimulate growth ( Table 1 ), clearly implicating the Tbx4 repressor activity in determination of HL identity. Ancestral Tbx4/5 is devoid of repressor activity A recent report indicated that the amphioxus Tbx4/5 ancestral gene shares FL growth stimulatory properties with Tbx4 and Tbx5 [15] . It was thus interesting to test whether conservation of growth activity is correlated with transcriptional activation. The full-length amphiTbx4/5 exhibited activator properties similar to Tbx5 ( Fig. 5a ), and this activity was mapped to amphiTbx4/5 C-terminus ( Fig. 5d ). Further, sequence comparisons suggest significant amino acid conservation within the amphioxus region homologous to the mouse activator domains (37% compared with 25% for the entire C-terminus, Fig. S1c,d ). These data are consistent with a model in which the growth stimulatory and activator properties of Tbx4/5 are more evolutionarily ancient compared with the repressor activity of Tbx4 that correlates with HL specificity. Contrary to the current view, the present work shows that Pitx1 -dependent Tbx4 is the primary effector of HL identity. This conclusion is supported for both skeletal and muscle patterning ( Table 1 ). This property is not shared by Tbx5, although both transcription factors share growth-promoting activities as previously reported [12] . Molecular dissection of Tbx4 and Tbx5 defined conserved transcriptional activation domains ( Fig. 6a ) that are correlated with their shared growth-promoting activity ( Fig. 6b ). The conservation of this activity and that of the growth-promoting activity in the evolutionary distant amphioxus Tbx4/5 support this model [15] . Significantly, previous gain-of-function paradigms used to investigate Tbx4 and Tbx5 only revealed this shared activity [12] . It seems that the HL-specific cell context is required to elicit the Tbx4 repressor activity that is correlated with its HL-specifying activities. The Tbx4 repressor domain mapped in the present work and inactivated by a human small-patella syndrome TBX4 mutation thus provides a molecular basis for HL specificity ( Fig. 6b ). The difficulty of revealing this Tbx4 activity in mouse FL gain-of-function experiments [12] , [20] may be due to the requirement for an HL-restricted co-repressor ( Fig. 6b ); expression of this co-repressor (or a related one) may not be as restricted in chicks, in which Tbx4 seemed to be sufficient to convey HL features to FL [9] . Further, the need for Pitx1 , together with Tbx4 , to alter mouse FL identity [12] may also be explained by Pitx1 -dependent expression of this putative co-repressor ( Fig. 6b ). 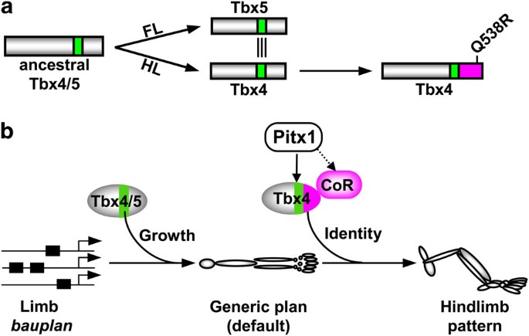Figure 6: Transcriptional basis for evolution of Tbx4/5 roles in limb development. (a) Schematic representation for divergence of an ancestral Tbx4/5 transcription factor that had activator domain (green) and for gain of repressor domain (magenta) in Tbx4. The small-patella syndromeTbx4mutation Q538R is within this domain. (b) The shared activator domain (green) is proposed to have an effect on limb bud growth, whereas the Tbx4 repressor domain (magenta) determines hindlimb identity. Expression ofTbx4in hindlimbs is enhanced byPitx1; similarly, expression of a putative co-repressor (CoR) required for Tbx4 repressor activity may be regulated byPitx1. Figure 6: Transcriptional basis for evolution of Tbx4/5 roles in limb development. ( a ) Schematic representation for divergence of an ancestral Tbx4/5 transcription factor that had activator domain (green) and for gain of repressor domain (magenta) in Tbx4. The small-patella syndrome Tbx4 mutation Q538R is within this domain. ( b ) The shared activator domain (green) is proposed to have an effect on limb bud growth, whereas the Tbx4 repressor domain (magenta) determines hindlimb identity. Expression of Tbx4 in hindlimbs is enhanced by Pitx1 ; similarly, expression of a putative co-repressor (CoR) required for Tbx4 repressor activity may be regulated by Pitx1 . Full size image The involvement of two key regulatory transcription factors, Pitx1 and Tbx4, in specification of HL identity (in contrast to the relatively minor role of Tbx5 in FL) provides molecular support to the idea that HL represents a novel plan compared with FL or a default bauplan ( Fig. 6 ). The shared growth-promoting activity of Tbx4 and Tbx5 is a likely critical component of this bauplan [11] , [35] . The repressor activity/domain of Tbx4 may thus be an evolutionary novelty. The gain of this Tbx4 repressor domain ( Fig. 6a ) may have led to the appearance of HL specificity, although it cannot be formally excluded that this feature was rather lost in the evolution of the Tbx5 and FL programme. Be that as it may, the Tbx4 repressor domain clearly provides a molecular basis for determination of HL identity ( Fig. 6b ). Posterior mesoderm expression of Pitx1 and that of the downstream Tbx4 thus result in HL-specific modulation of the generic limb programme. It was suggested and recently shown that changes in Pitx1 regulatory sequences are responsible for pelvic fin reductions in sticklebacks [22] , [24] and for loss of HL in manatees [36] . Although the gain of Pitx1 regulatory control is critical for specification of HL identity, the acquisition of a Tbx4 repressor domain/activity is also essential for execution of an HL-specific programme. It is thus likely that changes in both coding and regulatory sequences were needed for evolution of the posterior limbs. Mouse lines, embryos and skeletal preparations The Pitx1−/− mice were described previously [17] . Prx1-Tbx4 , Prx1-Tbx4Q538R and Prx1-Tbx5 transgenes were constructed using the Prx1 promoter (2.4 kb from −1,748 to +572 bp, graciously provided by Dr J.F. Martin) described by Martin and Olson [37] to drive the expression of mouse Tbx4 , Tbx4Q538R or Tbx5 full-length cDNAs, followed by SV40 polyadenylation sequences. Embryos were genotyped by PCR as described [17] using DNA isolated from the umbilical cord/amniotic membrane and a forward primer in the Prx1 enhancer (5′-CCAAAGGGGCTCTCTCCTTA-3′) with a reverse primer either in Tbx4/Tbx4Q538R (5′-CCCACCTTGATGTTCTCGAT-3′) or in Tbx5 (5′-GACCTGTCTTGGAATCAGG-3′) cDNAs. All mice used in this study were in a mixed genetic background. The noon of the day on which a vaginal plug was detected was staged as e0.5. Tbx4/Tbx4Q538R- or Tbx5-expressing Pitx1−/− embryos ( Pitx1−/− ; Prx1-Tbx4 , Prx1-Tbx5 or Prx1-Tbx4Q538R ) were obtained by crossing Pitx1+/− ; Prx1-Tbx4 , Prx1-Tbx4Q538R or Tbx5 males with Pitx1+/− females. For skeletal preparation, embryos staged as e17.5 were processed using a standard alcian blue and alizarin red staining procedure [21] . All animal procedures were approved and conducted in accordance with IRCM Animal Ethics Review Committee regulations. Bone length and angle measurements Limb bone length and calcaneus angle measurements were determined using the Northern Eclipse software, by averaging the indicated number of independent measurements on three different pictures of skeletal preparations laid on an agarose bed, taken so that the analysed bone sits in plane. Femur/humerus lengths were measured from head to the most distal point of the medial epicondyle. Tibia and fibula lengths were measured from their apex to the most distal malleolus extremity. Ulna and radius were measured from the styloid process to the olecranon or head, respectively. Pictures were taken on a dissecting scope (Leica MZ12) using a camera obtained from QImaging (Micropublisher 3.3 RTV). Statistical analyses Ratio of fibula/tibia bone length was compared using two-tailed Student's t -test. Whole-mount in situ hybridization and immunochemistry Whole-mount in situ hybridization and immunochemistry were performed as described [21] . Affinity-purified Tbx4 rabbit polyclonal antibodies raised against the maltose-binding protein fused to amino acids 327–390 of mTbx4 were used for Tbx4 immunohistochemistry. Whole-mount immunodetection [38] of MHC was performed on e14.5 embryos. Briefly, embryos were bleached in 5% H 2 O 2 , blocked in PBSMT (0.0038 M NaH 2 PO 4 , 0.0162 M Na 2 HPO 4 , 0.150 M NaCl, 2% milk, 2.5% Triton X-100 (pH 7.4)) and incubated with the monoclonal alkaline phosphatase-conjugated anti-MHC diluted 1/100 in PBSMT (MY32 clone; cat. no. A4335, Sigma). After numerous washes in PBSMT first and then in NTMT (0.1 M NaCl, 0.1 M Tris (pH 9.5), 0.050 M MgCl 2 and 0.1% Tween-20), alkaline phosphatase activity was revealed in NTMT using nitro blue tetrazolium/5-bromo-4-chloro-3-indolyl-phosphate substrate (Roche). MHC-stained HL muscles were identified by comparison [28] , [39] with data deposited at http://www.nimr.mrc.ac.uk/3dlimb/ using J Atlas View and generated by optical projection tomography [25] , [26] . Branchiostoma floridae (amphioxus) Tbx4/ 5 cDNA cloning AmphiTbx4/5 was cloned from 48-h embryonic cDNA (gift of Vincent Laudet and Hector Escriva, Lyon, France) by PCR using forward primer 5′-ATGTCTGGGGATTTGAAGGA-3′ and reverse primer 5′-TTATTGTGGAATTTGCATGG-3′ (from accession no. EU084005 ). Transfections The CV-1 cells were transfected by the calcium phosphate co-precipitation method. Cells (40,000) were plated in 12-well plates. A total of 3 μg of DNA (1.5 μg reporter plasmid, 0–0.75 μg effector plasmid or empty expression vector, 25 ng of CMV-β-galactosidase as internal control and 0–0.75 μg carrier pSP64 DNA) was used for each transfection, performed in duplicates. TBE-Luc and 5xUAS-Luc reporter plasmids were used [40] , [41] . Limb bud-derived cells were isolated from e11.5 CD1 mouse embryos by collagenase treatment (0.1%; Worthington), plated in 12-well plates (50,000 per well) and transfected using the Effectene reagent (Qiagen). A volume of 0.3 μg of DNA (100 ng reporter plasmid, 0–100 ng effector plasmid, 20 ng of CMV-β-galactosidase and 80 ng of pSP64 DNA) was transfected with 6 μl of Effectene reagent and 2.4 μl of enhancer, according to the manufacturer's recommendations. At 16 h after transfection, media were changed and cells were collected 24 h later, using lysis buffer (0.1 M Tris (pH 8.0), 0.5% Nonidet P-40 and 1 mM dithiothreitol). Luciferase and β-galactosidase activities were assayed in lysates with a luminometer using the luciferin substrate (Gold biotechnology) or the Galacto-Light system (TROPIX) [42] . Expression analysis Transgene expression was measured in dissected e11.5 HL buds that were frozen before RNA extraction using the RNeasy mini Kit following the manufacturer's instructions (Qiagen). cDNA synthesis was performed using SuperScriptIII Reverse Transcriptase (Invitrogen) and oligo-dT on 25 ng of total RNA. Quantitative real-time–PCR (MX-3005; Stratagene) was performed with cDNA and the SYBR Green kit (Qiagen). The following primers were used: Tbx4fwd (5′-ACAACAAATGGATGGTCGCAGG-3′) with Tbx4rev (5′-TTCTCGTCGGCCTTAACGATGT-3′) and Tbx5fwd (5′-GTACCAGTGTGAGAATGGTGTC-3′) with Tbx5rev (5′-CGACTCTGTCCTGTAAGAGGTA-3′). Tbx5 expression was never detected in Pitx1+/+ or Pitx1−/− HL. Relative expression was calculated relative to a control sequence within the glyceraldehyde 3-phosphate dehydrogenase ( Gapdh ) gene (primer GAPDHfwd (5′-TGCAGTGGCAAAGTGGAGAT-3′) with GAPDHrev (5′-ACTGTGCCGTTGAATTTGCC-3′)); its expression is unaltered in Pitx1−/− e11.5 HL buds. Western blot Hindlimb buds were dissected at e11.5 and kept at −80 °C during the genotyping procedure. Protein extracts were obtained by homogenization in lysis buffer (25% glycerol, 420 mM NaCl, 1.5 mM MgCl 2 , 0.2 mM EDTA, 20 mM HEPES (pH 7.9) and 5 mM PMSF, 1 μg ml −1 pepstatin, 1 μg ml −1 leupeptin, 1 μg ml −1 aprotinin and 1 mM dithiothreitol). Homogenates were submitted to three cycles of dry-ice freezing/thawing. Protein concentration was determined with Protein Assay Reagent Concentrate reagent (Bio-Rad) and 50 μg samples were separated by SDS–polyacrylamide gel electrophoresis and transferred onto polyvinylidene fluoride membranes. Blotting was first performed with the Tbx4 antibody; after stripping (100 mM of 2-mercaptoethanol, 2% SDS, 62.5 mM Tris–HCl (pH 6.7) for 30 min at 50 °C), membranes were blotted with the α-tubulin antibody (Santa Cruz, cat. no. sc-32293). Protein amounts were quantitated using ImageQuant 5.0 (Molecular Dynamics). How to cite this article: Ouimette, J.-F. et al . Divergent transcriptional activities determine limb identity. Nat. Commun. 1:35 doi: 10.1038/ncomms1036 (2010).